Visualizing the microscopic coexistence of spin density wave and superconductivity in underdoped NaFe1−xCoxAs Although the origin of high temperature superconductivity in the iron pnictides is still under debate, it is widely believed that magnetic interactions or fluctuations have a crucial role in triggering Cooper pairing. A key issue regarding the iron pnictide phase diagram is whether long-range magnetic order can coexist with superconductivity microscopically. Here we use scanning tunnelling microscopy to investigate the local electronic structure of underdoped NaFe 1− x Co x As near the spin density wave and superconducting phase boundary. Spatially resolved spectroscopy directly reveals both the spin density wave and superconducting gaps at the same atomic location, providing compelling evidence for the microscopic coexistence of the two phases. The strengths of the two orders are shown to anti-correlate with each other, indicating the competition between them. This work implies that Cooper pairing in the iron pnictides can occur when portions of the Fermi surface are already gapped by the spin density wave order. Similar to the cuprates, heavy fermions and organic superconductors, the iron pnictides also exhibit a superconducting (SC) phase emerging from a magnetically ordered parent state [1] , [2] . It is widely believed that magnetic interactions or fluctuations have a crucial role in mediating the iron-based high T C (critical temperature) superconductivity. Therefore, the evolution between the spin density wave (SDW) and SC phases in the underdoped regime of the phase diagram has attracted strong interests. A key question here is whether the magnetic order and superconductivity can coexist microscopically or mutually exclude each other. So far the available experimental methods used to answer this question are either spatially averaged probes or local ones without control of probing position, thus a consensus is still lacking [3] , [4] , [5] , [6] , [7] , [8] , [9] . Experiments on various iron pnictide compounds have revealed at least three categories of behaviour. Muon spin relaxation (μSR) and Mössbauer spectroscopy on LaFeAsO 1− x F x suggest that the abrupt transition from SDW to SC is first-order-like without coexistence of the two phases [4] . On the contrary, μSR on SmFeAsO 1− x F x (ref. 5 ) and BaFe 2− x Co x As 2 (ref. 8 ), together with nuclear magnetic resonance [6] and neutron scattering [7] on similar compounds, reveal the coexistence of the two phases. In an intermediate case, neutron scattering in CeFeAsO 1− x F x reveals a continuous transition, but the SDW and SC regimes only touch at a quantum critical point [3] . With its atomic scale structural and spectroscopic imaging capabilities, scanning tunnelling microscopy (STM) is an ideal probe for resolving the issue of microscopic phase coexistence in complex materials. In high T C cuprates, for example, STM has revealed the microscopic coexistence and distinct temperature/doping/spatial evolutions of the pseudogap and SC phases [10] , [11] . In the iron pnictides, however, there is no STM report so far regarding the relationship between the SDW and SC phases [12] . The main obstacle lies in the difficulty of identifying the spectroscopic feature of the SDW phase, namely the SDW gap, in STM studies of the iron pnictides. Recently, the SDW gap was directly observed in the 111-type NaFeAs parent compound owing to its excellent cleavage properties [13] . This progress makes the electron doped NaFe 1− x Co x As a promising candidate for investigating the evolution between magnetism and superconductivity in the underdoped regime. Here, we report STM studies of the local electronic structure of an underdoped NaFe 1− x Co x As near the SDW and SC phase boundary. Spatially resolved spectroscopy directly reveals both SDW and SC gap features at the same atomic location, providing compelling evidence for the microscopic coexistence of the two phases. The strengths of SDW and SC features are shown to anti-correlate with each other, indicating the competition of the two orders. The underlying physical picture is that Cooper pairing in the iron pnictides can occur when portions of the Fermi surface (FS) are already gapped by the SDW order. The regime T C < T < T SDW thus shows a strong resemblance to the pseudogap phase of the cuprates where growing experimental evidences suggest a FS reconstruction due to certain density wave order [14] , [15] , [16] . 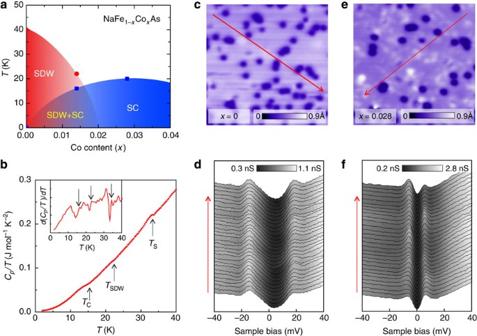Figure 1: Phase diagram of NaFe1−xCoxAs and STM results on parent and optimally doped samples. (a) Schematic electronic phase diagram of NaFe1−xCoxAs in the underdoped regime. The solid symbols mark the SDW and SC transition temperatures of parent (x=0), underdoped (x=0.014), and optimally doped (x=0.028) samples. (b) Temperature dependence of the specific heat and its derivative (inset) of the underdoped sample show the structural, SDW and SC phase transitions. (c) Constant current image of the cleaved surface of parent NaFeAs. (d) ThedI/dVspectroscopy taken on the parent compound along the red line in (c). There is a single p–h asymmetric SDW gap that is uniformly distributed in space. (e) Topography of the optimally doped sample, which shows more disorders due to Co doping. (f) ThedI/dVspectroscopy taken on the optimally doped sample along the red line in (e) shows a single p–h symmetric SC gap that is also quite homogeneous. Both images consist of 256 × 256 pixels taken on an area of 300 × 300 Å2. STM studies on the parent and optimally doped NaFe 1− x Co x As Figure 1a displays the phase diagram of the NaFe 1− x Co x As system in the underdoped regime around the SDW and SC phase boundary [17] . The solid symbols in the phase diagram represent the SDW and SC transition temperatures of the three samples studied here. The parent compound ( x =0) has a SDW phase transition at T SDW =40 K, and the optimally doped sample ( x =0.028) has a bulk SC transition at T C =20 K. The underdoped sample that lies in the middle ( x =0.014) is the most interesting one, which shows a structural transition at T S =32 K, a SDW transition at T SDW =22 K and a SC transition at T C =16 K. The three successive transitions are clearly manifested in the specific heat data shown in Fig. 1b and the resistivity results reported previously [17] . The main goal of our STM studies here is to determine whether the SDW-SC coexistence is microscopic or not. Figure 1: Phase diagram of NaFe 1− x Co x As and STM results on parent and optimally doped samples. ( a ) Schematic electronic phase diagram of NaFe 1− x Co x As in the underdoped regime. The solid symbols mark the SDW and SC transition temperatures of parent ( x =0), underdoped ( x =0.014), and optimally doped ( x =0.028) samples. ( b ) Temperature dependence of the specific heat and its derivative (inset) of the underdoped sample show the structural, SDW and SC phase transitions. ( c ) Constant current image of the cleaved surface of parent NaFeAs. ( d ) The dI/dV spectroscopy taken on the parent compound along the red line in ( c ). There is a single p–h asymmetric SDW gap that is uniformly distributed in space. ( e ) Topography of the optimally doped sample, which shows more disorders due to Co doping. ( f ) The dI/dV spectroscopy taken on the optimally doped sample along the red line in ( e ) shows a single p–h symmetric SC gap that is also quite homogeneous. Both images consist of 256 × 256 pixels taken on an area of 300 × 300 Å 2 . Full size image Figure 1c are the topographic images of the parent and optimally doped NaFe 1− x Co x As. Figure 1d display the dI/dV curves taken at the base temperature T =5 K along the red lines drawn in the topography. The measured dI/dV ( V , r ) is proportional to the local electron density of state (LDOS) at sample bias V and location r . As has been reported before, the parent compound exhibits a large, particle–hole (p–h) asymmetric SDW gap [13] . The optimally doped sample, on the other hand, shows a p–h symmetric SC gap with sharp coherence peaks. In either sample there is only one gap feature in the dI/dV curves. This, plus the fact that the dI/dV curves are spatially uniform despite the disorders in topography, suggest the existence of a single homogeneous phase for the parent and optimally doped samples. The distinct features of the SDW and SC gaps shown here provide the necessary fingerprints for identifying these two orders in the underdoped sample. 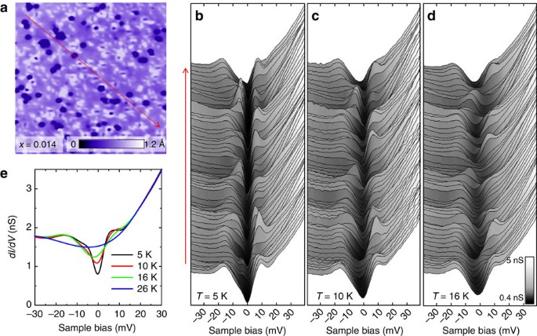Figure 2: ThedI/dVspectra of the underdoped NaFe1−xCoxAs. (a) A large area topography (600 × 600 Å2, 512 × 512 pixels) of the underdopedx=0.014 sample taken withV=100 mV andI=20 pA. (b) ThedI/dVspectra taken atT=5 K along the red line drawn in (a). The spectra are much more complex than that in the parent and optimally doped samples. They present strong spatial variations, and in most spectra there are clearly two-gap features at the same atomic location. (c,d) The same linecut spectra taken atT=10 K and 16 K, respectively. The small gap features become significantly weaker at 10 K and vanish completely at 16 K, indicating that it is the SC gap. The large gap persists to 16 K and shows the p–h asymmetric lineshape characteristic of the SDW gap. (e) The spatially averageddI/dVcurves taken at different temperatures, showing the evolution from the two-gap structure at 5 K to a single SDW gap at 16 K to the gapless normal state atT=26 K. The 26 K data are taken at the same area as those at low temperatures, but are not at exactly the same atomic locations. Coexistence of SDW and SC phases in underdoped NaFe 1− x Co x As Figure 2a shows a large-scale topography of the underdoped x =0.014 sample measured with sample bias V =100 mV and tunnelling current I =20 pA. Figure 2b shows the dI/dV curves measured at T =5 K along the line drawn in Fig. 2a . There are two striking differences between the spectroscopy in this underdoped sample and that shown above in the parent and optimally doped samples. First, most dI/dV spectra clearly exhibit two distinct gap features, a small p–h symmetric gap near the Fermi energy ( E F ) and a larger p–h asymmetric gap further away from E F . Second, the dI/dV curves display much more pronounced spatial variations. Both the size of the two gaps and amplitude of the gap edge peaks vary considerably from place to place. With increasing T to 10 K ( Fig. 2c ), the smaller gap becomes much shallower whereas the change of the larger gap is less significant. As T is increased further to 16 K ( Fig. 2d ), the T C of this sample, the small gap totally vanishes, indicating it is the SC gap. In contrast, the large gap remains and shows the p–h asymmetric lineshape characteristic of the SDW gap. Figure 2: The dI/dV spectra of the underdoped NaFe 1− x Co x As. ( a ) A large area topography (600 × 600 Å 2 , 512 × 512 pixels) of the underdoped x =0.014 sample taken with V =100 mV and I =20 pA. ( b ) The dI/dV spectra taken at T =5 K along the red line drawn in ( a ). The spectra are much more complex than that in the parent and optimally doped samples. They present strong spatial variations, and in most spectra there are clearly two-gap features at the same atomic location. ( c , d ) The same linecut spectra taken at T =10 K and 16 K, respectively. The small gap features become significantly weaker at 10 K and vanish completely at 16 K, indicating that it is the SC gap. The large gap persists to 16 K and shows the p–h asymmetric lineshape characteristic of the SDW gap. ( e ) The spatially averaged dI/dV curves taken at different temperatures, showing the evolution from the two-gap structure at 5 K to a single SDW gap at 16 K to the gapless normal state at T =26 K. The 26 K data are taken at the same area as those at low temperatures, but are not at exactly the same atomic locations. Full size image Figure 2e displays the spatially averaged dI/dV curves taken at four different temperatures, which clearly demonstrate the evolution from a two-gap structure at T =5 K to a single SDW gap at T =16 K. At T =26 K, that is, above the SDW transition temperature of this sample, both gaps are closed and the sample enters a rather conventional normal state. Thus, for temperatures between the SDW and SC phase transitions, the FS is partially gapped by the SDW order with a residual FS susceptible for Cooper pairing (there is a large residual DOS near zero bias even in the SDW phase of parent NaFeAs [13] ). This strongly resembles the phenomenology of the pseudogap phase in the cuprates. The SC gap features can be made clearer when the dI/dV curves below T C are divided by that measured at T C [10] . Shown in Fig. 3a are such normalized dI/dV curves where the data taken at T =5 K are divided by the 16 K ones at the same location. It is evident that the sharp, p–h symmetric SC gap is present in all the spectra. The averaged spectrum in Fig. 3b shows that the two coherence peaks are located at ±5 mV. If we use the distance between the two peaks to estimate the SC gap (note that the life time and thermal broadening effects are not considered in this rough criteria), then the gap size is around 2Δ SC =10 meV. The normalized 10 K dI/dV curves in Fig. 3c show that the SC gap is still present everywhere, although the gap depth is reduced by thermal excitations ( Fig. 3d ). The existence of the SC gap at every location of the sample demonstrates that superconductivity is a homogeneous rather than a filamentary phenomenon in this underdoped sample. The direct observation of both the SDW and SC gaps at the same atomic location, plus the fact that the sample exhibits both long-range SDW order and 100% SC volume fraction [17] , provide compelling evidence for the microscopic coexistence of the two orders. This coexisting state exhibits an averaged SDW gap 2Δ SDW =26 meV and SC gap 2Δ SC =10 meV intermediate between those of the parent (2Δ SDW =33 meV) and optimally doped (2Δ SC =11 meV) compounds. 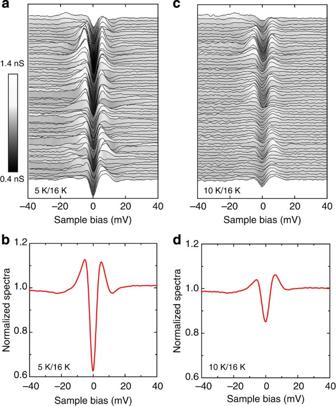Figure 3: The SC gap extracted by the normalization. (a) ThedI/dVcurves taken at 5 K are divided by that taken at the same location at 16 K. The SC gap feature is present in every location of the sample, indicating it is a bulk phase. (b) The spatially averaged spectrum shows that the coherence peaks are located atV=±5 mV. (c) Normalized spectra and (d) its spatial average of the 10 KdI/dVcurves. The SC gap features are still present everywhere although the gap is significantly filled by thermal excitations. Figure 3: The SC gap extracted by the normalization. ( a ) The dI/dV curves taken at 5 K are divided by that taken at the same location at 16 K. The SC gap feature is present in every location of the sample, indicating it is a bulk phase. ( b ) The spatially averaged spectrum shows that the coherence peaks are located at V =±5 mV. ( c ) Normalized spectra and ( d ) its spatial average of the 10 K dI/dV curves. The SC gap features are still present everywhere although the gap is significantly filled by thermal excitations. Full size image Competition between the SDW and SC phases Now the microscopic coexistence of the SDW and SC orders is unambiguously demonstrated, the next question is the interplay between them. We answer this question by studying the dI/dV curves in further details. 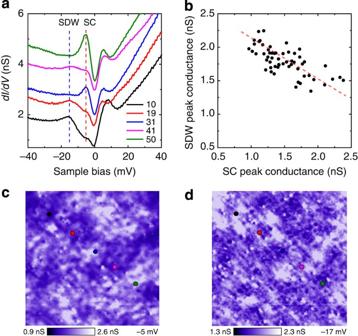Figure 4: Anti-correlation between the SDW and SC features. (a) Close-up of five representativedI/dVcurves taken at the locations marked in (c,d). The two-gap features are more pronounced in the negative bias side where the SDW gap has a gap edge peak at −17 mV and SC gap has a coherence peak at −5 mV. (b) ThedI/dVvalue at −17 mV as a function of that at −5 mV for all the curves inFig. 2b. There is an obvious anti-correlation between the two quantities indicated by the red broken line, which can also be seen directly in the five curves in (a). (c,d) ThedI/dVmaps (128 × 128 pixels in each one) measured at −5 mV and −17 mV on the same field of view asFig. 2a. The brightness of the two maps, which corresponds to the strength of SC and SDW phases, shows clear anti-correlation. Figure 4a zooms into five representative dI/dV curves taken at locations with nearly equal spacing along the line in Fig. 2a and marked in Fig. 4c . First we note that the two distinct gap features are more pronounced for negative bias, where the hump at V =−17 mV (marked by blue broken line) is associated with the SDW gap edge and that at V =−5 mV (red broken line) is associated with the SC gap edge. Second, when the −17 mV hump is more pronounced, such as in curve 10, 19 and 41, the SC coherence peak at −5 mV is strongly suppressed. On the contrary, in curve 31 and 50 the SC coherence peaks are very sharp, but the SDW hump at −17 mV becomes very weak. Therefore, there exists an obvious anti-correlation between the strength of the SDW and SC gap features. Figure 4b plots the dI/dV @−17 mV as a function of dI/dV@ −5 mV for all the curves shown in Fig. 2b , which clearly demonstrates the anti-correlation between the two quantities. Hence, the SDW and SC orders are shown to compete with each other. Figure 4: Anti-correlation between the SDW and SC features. ( a ) Close-up of five representative dI/dV curves taken at the locations marked in ( c , d ). The two-gap features are more pronounced in the negative bias side where the SDW gap has a gap edge peak at −17 mV and SC gap has a coherence peak at −5 mV. ( b ) The dI/dV value at −17 mV as a function of that at −5 mV for all the curves in Fig. 2b . There is an obvious anti-correlation between the two quantities indicated by the red broken line, which can also be seen directly in the five curves in ( a ). ( c , d ) The dI/dV maps (128 × 128 pixels in each one) measured at −5 mV and −17 mV on the same field of view as Fig. 2a . The brightness of the two maps, which corresponds to the strength of SC and SDW phases, shows clear anti-correlation. Full size image This competition can be visualized directly by utilizing the spectroscopic imaging capability of STM. Shown in Fig. 4c are the dI/dV maps, that is, the spatial distribution of the electron LDOS, at −17 mV and −5 mV biases for the same field of view as in Fig. 2a . The bright (dark) colour represents large (small) LDOS. Except for some sporadic spots with strong impurity states, the bright area of the first map matches very well with the dark area of the second map, and vice versa. The anti-correlation between the two dI/dV maps presents a direct visualization of the competition between the SDW and SC orders. The competition between magnetism and superconductivity has also been reported before by neutron and X-ray diffraction [7] , infrared spectroscopy [6] and μSR [8] , [9] , [18] studies on underdoped 122 compounds. The direct visualization of the microscopic coexistence and competition between the SDW and SC orders in the underdoped regime puts strong constraints on the theoretical models for the iron-based superconductors. The usual reason for not believing the coexistence of a density wave order and superconductivity is because once the FS is gapped by the former the susceptibility toward Cooper pairing is strongly suppressed. For the pnictides it has been demonstrated both theoretically and experimentally that in the SDW ordered state there are residual FSs. However, the topology of these FSs is entirely different from that of the non-magnetic state. As our data have directly demonstrated that Cooper pairing develops when the sample is already partially gapped by the magnetic order, we are driven to the conclusion that Cooper pairing must be developed on top of the residual (magnetically reconstructed) FSs. Under such condition the usual kinematic argument (for magnetic fluctuation caused Cooper pairing) in the non-magnetic state could break down. For example in [19] it was shown that when the SDW ordering moment is large, the residual FSs consist of a hole pocket at the Brillouin zone centre and two kidney-shaped electron pockets slightly displaced from it along the SDW ordering wavevector on either side. For this topology, magnetic fluctuations at the usual ordering wavevector cannot even scatter electron between FSs. In this case it is reasonable to believe SDW order will completely suppress SC pairing. On the other hand for weak SDW ordering [19] shows a residual hole pocket at the Brillouin zone centre and two electron pockets at the zone face, whose centre momentum is perpendicular to the magnetic ordering wavevector. For this topology it is reasonable to believe magnetic fluctuations at wavevectors perpendicular to the ordering wavevector will cause Cooper pairing. Here, the magnetic order does not eliminate Cooper pairing and SDW and SC orders may reside on different sections of the FS [20] . Therefore, our STM results suggest that SC pairing here is most likely caused by magnetic fluctuations in a SDW phase with a small ordering moment, which has a reconstructed FS with favourable topology. This proposal is supported by the extremely small ordering moment of 0.09 μ B detected by neutron scattering in parent NaFeAs [21] . The underlying physics revealed here bears strong resemblance to the pseudogap phenomena in the cuprates. Although the exact origin of the cuprate pseudogap is still under much debate, in recent years there are growing evidences that it may represent certain density wave orders, such as charge density wave [10] , [14] , [15] , [16] or incommensurate antiferromagnetic orders [22] , [23] . In either case, the FS is already reconstructed in the pseudogap regime and the SC phase develops on the residual FSs at low T. The density wave and SC orders compete for FS sections but may coexist with each other in real space. Here in underdoped NaFe 1− x Co x As we demonstrate unambiguously that a SDW gap is present at T > T C . Upon cooling below T C the SC gap opens on the residual FSs (analogous to the ‘Fermi arcs’ in the cuprates), as has been discussed theoretically [24] , [25] , [26] . This important common feature between the pnictides and cuprates suggests that the competition between Cooper pairing and density wave order might be generic to strongly correlated electron systems. Microscopically this must mean bare repulsive (local) electron interaction tends to renormalize into effective interactions favoring Cooper pairing and spin/charge density wave order at low energies. Theoretically such two phase coexistence is allowed by the Ginzburg–Landau theory even when the two order parameters compete (so long as not too strongly) [25] . Sample growth High quality NaFe 1− x Co x As single crystals are grown by the self flux technique as described elsewhere [17] . NaAs precursor is firstly synthesized at 200 °C for 10 h, and then powders of NaAs, Fe and Co are mixed together according to the ratio NaAs: Fe: Co=4: 1− x : x . The mixture is placed in an alumina crucible and then sealed into an iron crucible. The samples are put in a tube furnace with inert atmosphere and melt at 950 °C for 10 h before slowly cooled down to 600 °C at a rate of 3 °C h −1 . The actual chemical composition of the single crystals is determined by X-ray energy dispersive spectroscopy. STM measurements The STM experiments are performed with a low temperature ultrahigh vacuum STM system. As the NaFe 1− x Co x As samples degrade in ambient air, the samples are mounted onto the sample holder in a glove box filled with Ar gas. The sample holder is quickly transferred into the load-lock chamber and then into the ultrahigh vacuum sample preparation chamber. The NaFe 1− x Co x As crystals are cleaved in si tu at T =77 K (the cleaving stage is cooled by liquid nitrogen) and then transferred immediately into the STM sample stage. An electrochemically etched polycrystalline tungsten tip is used in the experiments. The STM topography is taken in the constant current mode, and the dI/dV spectra are collected using a standard lock-in technique with modulation frequency f =423 Hz. Before the STM experiments on the samples, the tungsten tip is carefully prepared and calibrated as described elsewhere [27] . How to cite this article: Cai, P. et al. Visualizing the microscopic coexistence of spin density wave and superconductivity in underdoped NaFe 1− x Co x As. Nat. Commun. 4:1596 doi: 10.1038/ncomms2592 (2013).